Protruding knob-like proteins violate local symmetries in an icosahedral marine virus Marine viruses play crucial roles in shaping the dynamics of oceanic microbial communities and in the carbon cycle on Earth. Here we report a 4.7-Å structure of a cyanobacterial virus, Syn5, by electron cryo-microscopy and modelling. A Cα backbone trace of the major capsid protein (gp39) reveals a classic phage protein fold. In addition, two knob-like proteins protruding from the capsid surface are also observed. Using bioinformatics and structure analysis tools, these proteins are identified to correspond to gp55 and gp58 (each with two copies per asymmetric unit). The non 1:1 stoichiometric distribution of gp55/58 to gp39 breaks all expected local symmetries and leads to non-quasi-equivalence of the capsid subunits, suggesting a role in capsid stabilization. Such a structural arrangement has not yet been observed in any known virus structures. Marine viruses are the most abundant and diverse life forms in the oceans. They constitute >90% of the nucleic acid containing material in the oceans [1] . It has been estimated that, based on their population (~10 30 ), if they were stretched out end to end, they could span sixty galaxies [1] . Only in the past decade have we started understanding the complexity of oceanic microbial ecosystems and their impact on global ecosystems [2] . Marine viruses are major biomass contributors to bio-geochemical cycles on earth, being responsible for 20% of the biomass cycled in the oceans everyday [1] . Synechococcus and Prochlorococcus are the most abundant cyanobacteria in the oceans, fixing ~30% of CO 2 of the atmosphere through photosynthesis. The cyanophages, or phages infecting cyanobacteria, are key players in host genetic diversity and microbial community variability [2] . Their modes of infection and horizontal gene transfer introduce population selection pressure, which drives host–virus co-evolution [3] . Also, lateral gene transfer [4] during evolution is probably responsible for the strong phylogenetic similarity found between the cyanophages and the phages of enteric bacteria [5] . Not surprisingly, cyanophages are efficient reservoirs of both genetic diversity [1] and novel genes [6] . Despite their importance, studies of marine viruses/phages are both recent and limited. This is especially true in terms of understanding their capsid structure and function, limiting our understanding of their efficiency as infection agents. Capsid subunits have to be capable of assembling into a closed icosahedral procapsid to package double-stranded (ds)DNA, and then transform to the mature capsid lattice stable enough to contain and protect the highly compressed genome. To date, only the mature capsids of cyanophage P-SSP7, infecting Prochlorococcus , have been structurally determined at near atomic resolution [7] . Here we present the near atomic resolution structure of cyanophage Syn5, which infects Synechococcus , the dominant cyanobacteria in both the rich coastal and oligotrophic waters of the ocean. Syn5 is a dsDNA virus belonging to the Podoviridae family with a T7 bacteriophage-like genome organization. In an earlier study on the genomic characterization of Syn5 (ref. 6 ), a low-resolution electron cryo-microscopy (cryo-EM) analysis reported ‘knob’-like features in the icosahedral capsid, along with a short tail and unique horn-like structure. The knob-like proteins display a unique structural arrangement in the mature capsid, but are absent in the immature virion structure, also reported here. We show here that these knob-like proteins break all local symmetry in an overall icosahedral capsid shell of the mature virion. Our structural and bioinformatic analyses assign two candidate gene products to the knob-like densities. Together, the structures provide significant insight into the assembly and maturation of marine viruses. Structure of the mature virion The mature Syn5 cyanophage was imaged using a JEM3200FSC electron cryo-microscope (300 keV) at liquid nitrogen temperature, images were recorded on a Gatan 10K × 10K CCD (charge-coupled device) camera. 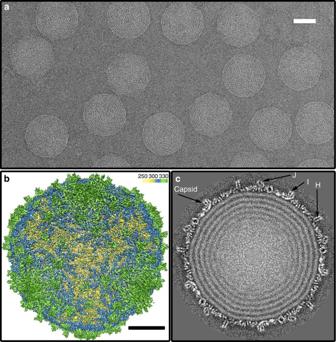Figure 1: Cryo-EM map of Syn5. (a) Syn5 virion particles observed in vitreous ice in various orientations. Scale bar, 300Å. (b) Icosahedral map of Syn5 at 4.7 Å coloured radially, shows the arrangement of pentamers (green), hexamers (blue) and protruding densities (green) forming the capsid structure. Scale bar, 150Å. (c) A 2D slice of the map showing the capsid wall and the protruding densities labelled as H, I and J. Figure 1a shows a typical image of Syn5. The power spectrum of Syn5 particles in an individual CCD frame [8] is shown in Supplementary Fig. 1a , indicating visible signal beyond 5 Å resolution. An ab initio featureless initial model ( Supplementary Fig. 1b ) was generated using a small set (~1,000) of particles by Fourier cross-common lines principle [9] implemented in multi-path simulated annealing three-dimensional (3D) reconstruction routine [10] . A final icosahedral reconstruction was obtained from ~12,000 individual particle images ( Fig. 1b ). The resolution of the map was estimated and validated by using the high-resolution (HR) noise substitution method [11] . A Fourier shell correlation (FSC true ) was calculated as described previously [11] estimating the resolution of the map to be 4.7 Å at 0.143 FSC cut-off ( Supplementary Fig. 1c ). Figure 1: Cryo-EM map of Syn5. ( a ) Syn5 virion particles observed in vitreous ice in various orientations. Scale bar, 300Å. ( b ) Icosahedral map of Syn5 at 4.7 Å coloured radially, shows the arrangement of pentamers (green), hexamers (blue) and protruding densities (green) forming the capsid structure. Scale bar, 150Å. ( c ) A 2D slice of the map showing the capsid wall and the protruding densities labelled as H, I and J. Full size image A characteristic feature of the map is the presence of 60 copies of hexameric capsomeres and 12 copies of pentameric capsomeres ( T =7). One striking feature of the hexameric capsomere, which is different from any known bacteriophage structure, is the presence of protruding densities ( Fig. 1b ) referred hereby as ‘knob-like proteins’ [6] . Figure 1c shows a slice view of the map with three such knob-like densities protruding at different heights from the capsid wall (labelled as H, I and J). Major capsid protein (gp39) of the mature virion At the reported resolution, the capsid density map clearly reveals the secondary structural elements (SSEs) of the protein subunits, such as long α-helices and large β-sheets [12] , [13] . On the basis of location, the presence of SSEs and the expected structural similarity to other known bacteriophage major capsid proteins ( Supplementary Fig. 2a,b ), such as HK97 (gp5) [14] , ε15 (gp7) [15] and T7 (gp10A) [16] , we segmented, averaged and constructed de novo Cα backbone models for each gp39 subunit in the asymmetric unit using Gorgon [17] . 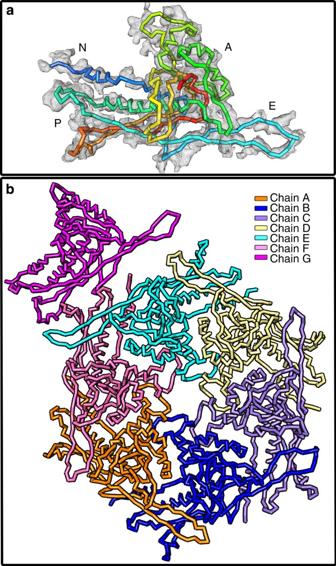Figure 2: Major capsid protein gp39. (a)De novobackbone model of gp39 fit in the corresponding map density (grey) shows an HK-97-like fold; the residues are coloured blue to red from the N- to the C-termini. (b) Backbone model of the seven chains A–G of gp39 in one asymmetric unit forming theT=7 icosahedral capsid. Figure 2a shows a model of one gp39 subunit superimposed on the density map; the major domains—A, P, E-loop and N-arm domains—are clearly evident, while model of one asymmetric unit with seven gp39 subunits (Chain A–G) is seen in Fig. 2b . To validate the model, an analysis of the uniqueness of the solution obtained for the Cα trace was carried out using an independent de novo modelling tool, Pathwalker (discussed in Methods section). Figure 2: Major capsid protein gp39. ( a ) De novo backbone model of gp39 fit in the corresponding map density (grey) shows an HK-97-like fold; the residues are coloured blue to red from the N- to the C-termini. ( b ) Backbone model of the seven chains A–G of gp39 in one asymmetric unit forming the T =7 icosahedral capsid. Full size image The major capsid protein of Syn5 (gp39) shows only ~16% sequence identity when compared with the major capsid proteins of HK97 (gp5) [14] and ε15 (gp7) [15] , whereas a higher sequence identity of ~44 and ~26% is observed with the coat proteins of P-SSP7 (gp10) [7] and T7 phage (gp10) [16] , respectively. In terms of structural domain arrangement, gp39 (332 aa) is topologically most similar to gp10A (345 aa), a coat protein of T7, and gp5 (282 aa), a coat protein of HK97. A Cα root mean squared deviation of ~2.3 Å is obtained from a pairwise topology comparison between gp39 and gp10A or gp5 with an overall ~115 matched residues in each case [18] . A couple of significant differences are found in the A-domain region of the above proteins. In Syn5, the coat protein gp39 shows the presence of an ‘extra’ loop (~30 aa, coloured yellow, Fig. 2a and Supplementary Fig. 3a ) when compared with gp5 in HK97. This loop region of gp39 subunits (chains C and D) are seen bound to protruding knob-like proteins (green densities, Fig. 3a ). Second, in gp39 the loop region (~26 aa) forming the opening at the local six-fold axis of the hexamer ( Fig. 2b ) is wider and orthogonal to that observed in case of gp5 (HK97), where this loop is elevated straight towards the centre of the hexamer ( Supplementary Fig. 3a ). A similar difference as above is observed on comparison of the hexameric gp39 subunits (chains A–F) with the pentameric gp39 subunit (chain G), where the A-domain loop of the hexameric subunits around the opening at the six-fold axis is tilted by a ~90° angle to that of the pentameric gp39 subunits lying around the five-fold axis ( Supplementary Fig. 3b ). 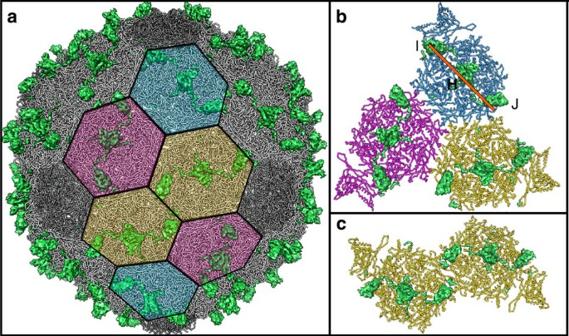Figure 3: Protruding knob-like densities. (a) An overall arrangement of the knob-like densities (green) protruding from the capsid surface (grey model) formed by the major capsid protein gp39, where the pentameric vertices are shown in dark grey. Two triangular (T) faces are annotated as blue, pink and yellow hexagons per T-face to show strict icosahedral three- and two-fold symmetry. (b) A view of the strict icosahedral three-fold showing the arrangement of the protruding densities (green). The three knob-like densities (green) are labelled such that I faces the vertex, while J faces the neighbouring hexamer and H lies at the centre of the hexamer. (c) A view of the strict icosahedral two-fold showing the relative arrangement of I/H/J. Figure 3: Protruding knob-like densities. ( a ) An overall arrangement of the knob-like densities (green) protruding from the capsid surface (grey model) formed by the major capsid protein gp39, where the pentameric vertices are shown in dark grey. Two triangular (T) faces are annotated as blue, pink and yellow hexagons per T-face to show strict icosahedral three- and two-fold symmetry. ( b ) A view of the strict icosahedral three-fold showing the arrangement of the protruding densities (green). The three knob-like densities (green) are labelled such that I faces the vertex, while J faces the neighbouring hexamer and H lies at the centre of the hexamer. ( c ) A view of the strict icosahedral two-fold showing the relative arrangement of I/H/J. Full size image A pairwise FSC analysis between the seven gp39 subunits of an asymmetric unit shows a higher correlation at lower frequencies between four hexameric subunits (chains B:E and C:F; green curves, Supplementary Fig. 3c ). These two FSC curves (green) show a higher than average FSC curve (solid black) when compared with the other subunit in a pairwise comparison (blue and red curves). These four gp39 subunits (chains B, C, E and F) are seen bound to the knob-like proteins, discussed later. Overall, their structural similarity is measured to be ~6.5 Å as measured by the FSC=0.33. The primary structure differences among the gp39 subunits lie in the A-domain and E-loop regions (red oval, Supplementary Fig. 3b ). For instance, the E-loop of the pentameric gp39 subunit is tilted by ~45° in comparison to the hexameric gp39 subunits, showing the poorest correlation. Protruding knob-like capsid proteins identified The mature capsid of Syn5 contains several knob-like major densities protruding from the capsid surface ( Fig. 3a ). Here the knob-like proteins are labelled as I/H/J based on their positioning along a diagonal across the hexameric capsomere ( Fig. 3b ). The density H is located at the centre of the hexameric capsomere. Both I and J are present at the two opposite ends of the diagonal such that protein I always faces the pentameric vertex, while J faces the neighbouring hexameric capsomere. As seen in Fig. 3b,c , these knob-like proteins follow the strict icosahedral two/three-fold symmetries as expected from an icosahedral reconstruction. These additional protruding densities were segmented after fitting the gp39 models to the density map. The segmented H density has a clip-like dimeric structure, labelled as H1/H2 in Fig. 4a–c . It shows elongated rod-like densities at the base near the six-fold (capsid-binding domain), while the top part flares outwards from the capsid surface (protruding domain) ( Fig. 4b ). Automatic segmentation of H using Segger19 (ref. 19 ) and a rotational symmetry analysis revealed that it is a dimer, with two monomeric subunits related by a two-fold symmetry normal to the capsid surface ( Fig. 4c and Supplementary Fig. 4a ). The capsid-binding domain of H1 and H2 further extends into densities running parallel to the capsid surface in four directions (grey densities, Fig. 4a ). The densities I and J appear to be anchored at the opposing ends of the diagonal formed by these elongating densities. 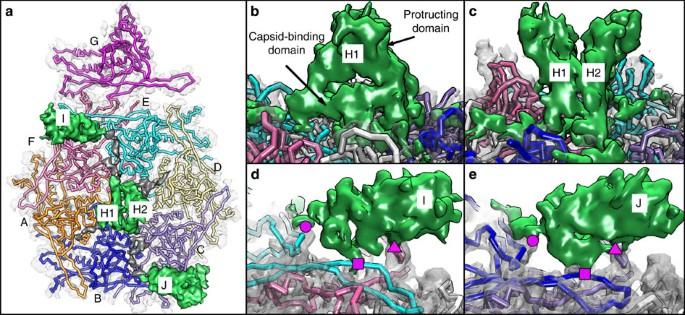Figure 4: Binding sites of I/H/J. (a) One asymmetric unit of Syn5 consisting of 11 polypeptide chains, labelled as A–J, where the two-polypeptide chains of H are labelled as H1/H2. The seven major capsid protein gp39 models (A–G) follow the colour scheme ofFig. 2b. Here the knob-like proteins (green) are seen connected by grey densities. (b) The binding site of the density H to gp39 (a side view such that only one monomer H1 is seen). (c) A close up of H in a 90° rotated view of (b) (a side view such that both monomers H1/H2 are seen). (d,e) A close up of the equivalent binding sites of densities I and J to gp39, annotated by magenta circle, square and rectangle symbols. Figure 4: Binding sites of I/H/J. ( a ) One asymmetric unit of Syn5 consisting of 11 polypeptide chains, labelled as A–J, where the two-polypeptide chains of H are labelled as H1/H2. The seven major capsid protein gp39 models (A–G) follow the colour scheme of Fig. 2b . Here the knob-like proteins (green) are seen connected by grey densities. ( b ) The binding site of the density H to gp39 (a side view such that only one monomer H1 is seen). ( c ) A close up of H in a 90° rotated view of ( b ) (a side view such that both monomers H1/H2 are seen). ( d , e ) A close up of the equivalent binding sites of densities I and J to gp39, annotated by magenta circle, square and rectangle symbols. Full size image The segmented densities for I and J appear globular, exhibiting similar size and shape ( Fig. 4d,e ). Superposition of the I and J, and a difference map analysis revealed only minor structural differences; a structural similarity of 7Å was observed between the segmented densities of I and J from the FSC analysis ( Supplementary Fig. 4b ). From the above analyses, we conclude that the densities observed at the I/J positions along each hexameric capsomere of the map are the same, which in turn suggests that they are made of the same protein. Both proteins I and J show three equivalent attachment sites (labelled with a circle, square and triangle in magenta, Fig. 4d,e ) to two gp39 subunits lying at the opposite ends of the diagonal (that is, chains E/F and B/C, respectively). Density I is attached at two sites of the same gp39 subunit (chain E), namely the loop region immediately after the long helix (circle) and at the end of the E-loop (square) ( Fig. 4d ). While at the other end, protein I extends further, slightly elevated, attaching to the protruding loop of the A-domain of the neighbouring gp39 subunit (triangle, chain F). Similarly, three equivalent attachment sites are observed for diagonally opposite protein J at two corresponding gp39 subunits (chain B/C) ( Fig. 4e ). This suggests that each of the I and J subunits spans across two adjacent gp39 subunits within a capsomere to stabilize the hexon. Gene product assignments to the knob-like proteins While assignment of the gp39 to the map density was straightforward because of expected phage capsid fold, the determination of corresponding gene products for I, J and H (H1/H2) was more challenging. Three late gene products, gp55 (156 aa), gp57 (131 aa) and gp58 (169 aa), were potential candidates [20] for the above densities. We performed several computational analyses on these candidates, both on their sequences and the map densities for I, J and H (H1/H2), including secondary structure prediction [21] , [22] , protein stability, amino-acid composition [23] , [24] and density-based secondary structure analysis with SSEHunter [25] . Sequence analyses predict [23] , [24] gp55 and gp58 to be stable proteins with consensus secondary structure predictions [21] , [22] , while gp57 is predicted to be an unstable protein with no consensus secondary structure prediction. Secondary structure element analysis with SSEHunter of densities I/J identified major β-sheet regions (blue sheets, Fig. 5a ), while density H1 or H2 showed two major helices in its capsid-binding domain (green cylinder, Fig. 5b ). The secondary structure prediction of gp55 (156 aa) revealed mostly β-strands and loops, while the gp58 showed three major helices (at N-terminus) along with strands/loops ( Fig. 5a,b ). On the basis of converging results from the above density and sequence-based structure predictions, a correspondence was established between gp55 and I/J densities, as well as gp58 and the H1/H2 density. Also, the density and sequence analysis together hint that gp58 (~169 aa) forms a dimer consisting of two polypeptide chains. Hence, we conclude that each hexameric capsomere of Syn5 has two copies of gp55 at respective I/J positions and two copies of dimeric gp58 at positions H1 and H2. Here we were able to locate the SSEs such as helices/sheets ( Fig. 5a,b ); however, we were not able to build a model due to insufficient resolvability of these protruding regions and lack of homologous structures in the PDB for gp55/58. 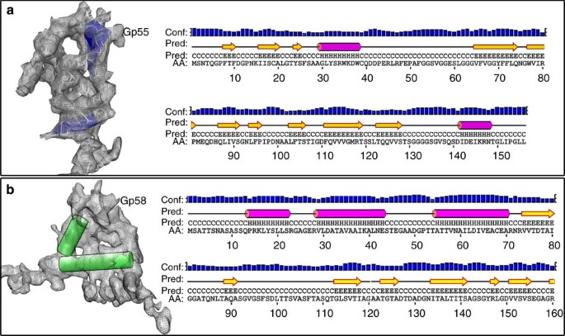Figure 5: SSEs in I/J and H1/H2. The figure shows (a) gp55 (I/J) and (b) gp58 (H1/H2). Both (a,b) on the left show the density-based localization of the SSEs (helices as green cylinders and β-sheets as blue sheets) for I/J and H1/H2 densities, respectively. Two helices annotated by green cylinders are predicted in the capsid-binding domain of H. On the right is seen a sequence-based secondary structure prediction for gp55 and gp58, the corresponding gene candidates for densities I/J and H1/H2, respectively. Here ‘Conf’ refers to confidence in the secondary structure prediction, where the height of the histogram relative to a scale (on the left and right ends) represents the confidence of prediction on a scale of 0–1 (low=0 and high=1) and ‘Pred’ refers to the predicted secondary structure for a region. Figure 5: SSEs in I/J and H1/H2. The figure shows ( a ) gp55 (I/J) and ( b ) gp58 (H1/H2). Both ( a , b ) on the left show the density-based localization of the SSEs (helices as green cylinders and β-sheets as blue sheets) for I/J and H1/H2 densities, respectively. Two helices annotated by green cylinders are predicted in the capsid-binding domain of H. On the right is seen a sequence-based secondary structure prediction for gp55 and gp58, the corresponding gene candidates for densities I/J and H1/H2, respectively. Here ‘Conf’ refers to confidence in the secondary structure prediction, where the height of the histogram relative to a scale (on the left and right ends) represents the confidence of prediction on a scale of 0–1 (low=0 and high=1) and ‘Pred’ refers to the predicted secondary structure for a region. Full size image A BlastP sequence analysis [26] of gp55 returns TonB-dependent receptors as top hits with 28% sequence identity. A multiple sequence alignment between gp55 and the top Blast hit result showed similarities with the region of TonB receptor belonging to the porin superfamily (aa 211–385) ( Supplementary Fig. 5 ). The TonB receptors play a role in sensing and signalling in the outer membrane of the Gram-negative bacteria and share a β-barrel-like structure [27] , [28] . The host of cyanophage Syn5 is also a Gram-negative cyanobacteria Synechococcous . Both gp55 sequence secondary structure prediction and density analysis hint towards a mostly β-stranded structure of gp55 ( Fig. 5a ), which might explain the observed sequence similarities with the TonB-dependent receptors (mostly β-stranded). Also, it is known that viruses can mimic both ligands and cell surface receptors of host cells, also known as the molecular mimicry mechanism [29] . Such a mechanism is used to parasitize the host cell surface receptors to hijack and affect certain cellular processes. It is possible that gp55 plays a role in weak host-cell surface recognition or increases the host-cell nutrient intake in a nutrient-deficient environment by mimicking the siderophore/TonB-dependent cell surface receptors and hence, increasing the efficiency of virus infection [29] . Sequence analysis of gp58 (169 aa) revealed 25% sequence identity with the Hoc protein [30] from T4. However, most of the observed sequence identity is randomly distributed over the four domains of the Hoc protein (400 aa). Both gp58 and Hoc proteins are observed at the six-fold opening of the hexamers in Syn5 and T4 capsids, respectively. The Hoc proteins exist as monomers, consisting of three of the four domains with antigenic Ig-like structure [31] , while gp58 is present as a dimer with no predicted Ig-like domains. From the sequence analysis of gp58 the N-terminus region is predicted to have major helices (16–18 residues long). In our map we also observe two ~30-Å long rod-like helical densities ( Fig. 5b ) at the capsid-binding domain of each monomer of gp58, anchored at the six-fold depression of the capsid surface. This would suggest that the N-terminus region of gp58 is most likely the capsid-binding domain, which in turn implies that the C-terminus (predicted to be mostly loops and strands) possibly forms the protruding domain. Symmetry breaks observed at all local interaction sites In the mature Syn5 virion, the major capsid protein gp39 has an icosahedral packing, but the presence of protruding knob-like proteins gp55/58 introduces asymmetric local interfaces among the neighbouring capsomere gp39 subunits. Such a distribution of the knob-like proteins across the icosahedral capsid is not observed in other known phage/virus structures. 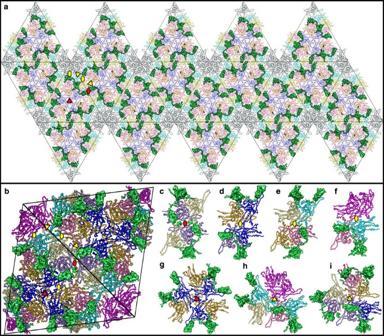Figure 6: Symmetry breaks in Syn5 icosahedral lattice. (a) A 2D representation of theT=7 lattice in Syn5, showing all the 20 triangular faces with an arrangement of the knob-like densities (green); the hexameric gp39 models are coloured as per colour scheme ofFig. 2b, while the pentameric gp39 is coloured grey. The strict icosahedral three- and two-fold symmetry axes between one set of two triangular (T) faces are marked by red triangle and oval symbols, respectively, while the local three- and two-fold axes are marked by corresponding yellow symbols. (b) A close up of two T-faces from (a) is shown enclosed in a rhombus shape (solid black lines). (c–f) An array of all the two-fold interfaces observed in Syn5, where (c) shows the strict icosahedral two-fold interface (axis, red oval) and (d–f) show the local two-fold interfaces (axes, yellow oval). (g–i) An array of all the three-fold interfaces, with (g) showing the strict icosahedral three-fold interface (axis, red triangle) and (h,i) showing the local three-fold interfaces (axes, yellow triangle). Figure 6 and Supplementary Movie 1 show a range of all such interfaces observed at both the strict and local two/three-fold symmetry interactions between the capsomere subunits. Figure 6: Symmetry breaks in Syn5 icosahedral lattice. ( a ) A 2D representation of the T =7 lattice in Syn5, showing all the 20 triangular faces with an arrangement of the knob-like densities (green); the hexameric gp39 models are coloured as per colour scheme of Fig. 2b , while the pentameric gp39 is coloured grey. The strict icosahedral three- and two-fold symmetry axes between one set of two triangular (T) faces are marked by red triangle and oval symbols, respectively, while the local three- and two-fold axes are marked by corresponding yellow symbols. ( b ) A close up of two T-faces from ( a ) is shown enclosed in a rhombus shape (solid black lines). ( c – f ) An array of all the two-fold interfaces observed in Syn5, where ( c ) shows the strict icosahedral two-fold interface (axis, red oval) and ( d – f ) show the local two-fold interfaces (axes, yellow oval). ( g – i ) An array of all the three-fold interfaces, with ( g ) showing the strict icosahedral three-fold interface (axis, red triangle) and ( h , i ) showing the local three-fold interfaces (axes, yellow triangle). Full size image In Fig. 6a , the complete Syn5 capsid is presented in a two-dimensional (2D) lattice form, showing all the quasi-equivalent sites for a T =7 capsid (red oval/triangle symbols for strict icosahedral two/three-fold, respectively, while yellow symbols for local two/three-fold sites). In Fig. 6b is shown a close up of two neighbouring triangular faces where the icosahedral strict and local symmetry axes are labelled as above. Four types of two-fold interfaces are observed between the gp39 subunits of neighbouring capsomeres ( Fig. 6c–f ). Here in addition to the strict icosahedral two-fold symmetry interface ( Fig. 6c ), three additional local two-fold interfaces are present between the gp39 subunits of neighbouring hexameric and hexameric/pentameric capsomeres ( Fig. 6d–f ). However, these local two-fold symmetries are broken due to the unique diagonal positioning of gp55/58 (I/H/J positions) in the asymmetric unit. Similarly, Fig. 6g–i shows the three types of three-fold interface observed between the gp39 subunits of neighbouring capsomeres. In Fig. 6f is shown the three-fold interface observed at the icosahedral strict three-fold axis. Two local three-fold interactions are present between the gp39 subunits of neighbouring hexameric and hexameric/pentameric capsomeres ( Fig. 6h,i , respectively), but the local three-fold symmetry is again broken due to the gp55/58 binding. Our structure of the mature virion of Syn5 presents for the first time a direct structural insight of a marine virus, Syn5, which infects the dominant cyanobacteria Synechococcous in the oceans. Surprisingly, in spite of being relatively primitive on an evolutionary scale, the structure of Syn5 reveals a unique and complex arrangement of capsid subunits not observed in other virus structures ( Supplementary Fig. 6 ). Here each asymmetric unit has four more knob-like capsid subunits (two copies of gp55 and two copies of gp58), in addition to the regular seven major capsid subunits (gp39) in a T =7 arrangement. Consequently, each asymmetric unit in Syn5 is made up of 11 polypeptide chains with a stoichiometric ratio of 7:2:2 for gp39:gp55:gp58. Such a non 1:1 distribution of gp55/58 to gp39 breaks all expected local symmetries in an overall icosahedral capsid shell. This in turn leads to non-quasi-equivalence of the capsid subunits, making the structural arrangement of Syn5 an exception to the theory of quasi-equivalence [32] . The studies of marine viruses are both recent and limited; here our structural analysis of Syn5 elucidates an understanding of their capsid structure and function. The mature capsid of dsDNA viruses need to be stable enough to resist the pressure for highly condensed genome [33] . In other phage/virus structures, the outer capsid proteins (also known as decoration/stabilizing/stapling proteins) are usually found at the three- or two-fold regions (dotted lines, Supplementary Fig. 6 ), with the three-fold known as the weakest site for icosahedral capsids [33] , [34] . In HK97, covalent bonding stabilizes the three-fold sites, although many phages/viruses recruit decoration proteins to stabilize this region. Phages lambda, L and T4 stabilize the three-fold region by incorporating trimers ( Supplementary Fig. 7 ) of stabilizing proteins, gpD [35] , Dec [36] and Soc [37] , respectively, while in adenovirus, minor capsid protein IX trimers are incorporated in this region [38] . In the case of ε15, the stapling protein gp10 is present as dimers, stabilizing the two-fold interactions between the neighbouring capsomeric subunits [15] ( Supplementary Fig. 7 ). The presence of penton base-associated fibre trimers in adenovirus [39] , [40] cause a symmetry break at the five-fold; however, unlike in Syn5, the symmetry at the quasi-equivalent local two/three-fold sites is maintained. While Syn5 contains a major capsid protein (gp39) similar to other bacteriophages, the two other knob-like outer capsid proteins (gp55/58) are novel proteins. Unlike the outer capsid proteins observed in viruses/phages mentioned above, these knob-like proteins (gp55/58) in Syn5 do not bind at the inter-capsomere interfaces located at the strict icosahedral or local two/three-fold symmetry axes ( Supplementary Fig. 7 ). Instead, both gp55/58 are bound to the major capsid (gp39) subunits in unique diagonal positions within a hexameric capsomere presumably, stabilizing the intra-capsomere hexameric subunit interactions ( Fig. 4d,e ). Furthermore, none of the pentameric subunits has any of these associated proteins. Again, such a structural arrangement of capsid proteins has never been observed in any icosahedral virus structure. An insight into the functional implications of the unique arrangement of outer capsid proteins observed in Syn5, is gained by a comparative analysis of the hexameric capsomeres, observed in known T =7 virus structures. In Syn5, the opening at the six-fold, composed of six gp39 proteins, measures ~28–30 Å in diameter, while the opening measures ~12–14 Å in other phages such as HK97 (ref. 14 ), ε15 (ref. 15 ), P22 (ref. 41 ) and P-SSP7 (ref. 7 ) ( Fig. 7a and Supplementary Fig. 2b ). This is due to a loop in the A-domain, which is orientated differently than the corresponding loop in other known phage structures ( Supplementary Fig. 3a ). Such a significantly wider opening at the six-fold in Syn5 would likely not provide the necessary protection of the viral genome. The positioning of the gp58 protein dimer (H1 and H2) atop the six-fold opening, together with its size relative to the six-fold axis opening, suggests that it is a plug that seals the wide opening, protecting the genome and enhancing capsid stability ( Fig. 7b,c ). Owing to the size and geometry of the pentameric opening, the gp58 dimer would not be able to fit the dimensions. A similar arrangement has been observed in T4 phages, where the outer capsid protein, Hoc, does not bind to the mutant hexamer opening when it is made up of only five major capsid (gp23) subunits [31] . 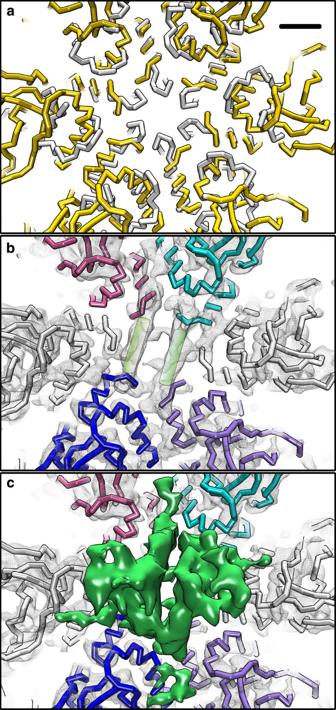Figure 7: Gp58 (H1/H2) incorporation. (a) Difference between the opening at the centre of the hexamer in Syn5 (gold) and that seen in HK97 (white). Scale bar, 13Å. (b) The same region of (a) in Syn5 map (slice view, grey mesh) with fitted Syn5 model (white). Here two helical densities (green cylinders) are observed connecting four gp39 subunits (coloured). (c) A non-slice view of (b) to illustrate that the helical densities in (b) correspond to the capsid-binding domain of gp58 (green) contributed by its H1 and H2 monomers. Figure 7: Gp58 (H1/H2) incorporation. ( a ) Difference between the opening at the centre of the hexamer in Syn5 (gold) and that seen in HK97 (white). Scale bar, 13Å. ( b ) The same region of ( a ) in Syn5 map (slice view, grey mesh) with fitted Syn5 model (white). Here two helical densities (green cylinders) are observed connecting four gp39 subunits (coloured). ( c ) A non-slice view of ( b ) to illustrate that the helical densities in ( b ) correspond to the capsid-binding domain of gp58 (green) contributed by its H1 and H2 monomers. Full size image Interestingly, two gp55s are always bound to the E-loop region of two gp39 subunits, which are also bound to the gp58 molecule at their A-domains. Such a specific binding explains the co-occurrence of two gp58 and two gp55 molecules always along one specific diagonal of a hexameric capsomere. This also hints that the incorporation of gp55 molecules is not solely guided by the curvature of the hexamer. Possibly the incorporation of gp58 dimer to seal the six-fold opening causes some domain movements, which in turn exposes binding sites for the incorporation of two gp55 molecules. This would mean that gp55 incorporation compensates for the conformational instability caused by gp58 binding. Such domain-level conformational changes induced by the binding of small proteins has been observed in other macromolecular complexes such as ribosomes, where the binding of ribosome modulation factor induces a conformational change in the 30S head domain of the 100S ribosome, exposing new interaction sites [42] . Our cryo-EM analysis of the procapsids of Syn5 show the absence of protruding densities corresponding to gp55/58 in the immature prohead particles, which instead have a thicker, less angular and smaller cage-like structure ( Supplementary Fig. 8a,b ). This hints at the incorporation of these outer capsid proteins in the later stage of maturation. The absence of protruding proteins in the procapsids may facilitate scaffolding protein release through the openings at the hexameric capsomeres [41] . It is known that the filling of DNA during the maturation process of the viruses can produce extreme pressures (~60 atm) causing capsid expansion, which in turn lead to structural rearrangements [33] . It is possible that such events in Syn5 lead to a wider opening at the six-fold axis of hexameric capsomeres, pushing the pentameric capsomeres upwards, as observed from the difference analysis between the procapsid and mature capsid maps ( Supplementary Fig. 8c ). As a result, gp58 may be added during maturation to seal the openings at the hexameric capsomeres and protect the viral genome. In turn, gp55 may also be added concurrently to help lock in the gp58 dimer, as discussed above. The expansion and angularization of the capsid may contribute to the availability of the binding sites along gp39 for both gp55 and gp58, explaining their incorporation along the same diagonal of the hexameric capsomeres. As such, both gp55 and gp58 appear to play the role of stabilizing proteins in the mature capsid of Syn5. Also, the sequence analysis of gp55 hints that it might play a role in weak host cell surface recognition or mimic host cell surface receptors. These cyanophage–host systems are found in harsh oligotrophic environments of the oceans [43] ; such surface proteins might help in binding to non-host cells as well [30] to aid in travelling to their widely separated host cells. Considering virus–host co-evolution [44] , cyanophages such as Syn5 are likely as ancient as their host cyanobacteria (~2.8 billion years), presenting an ancient lineage to the present day viruses. It is known that cyanophages such as Syn5 and P-SSP7 show synteny and homology to enteric phages [45] . Unlike Syn5, the marine virus P-SSP7 does not have accessory proteins to enhance capsid stability. However, some relatively more recent enteric phages and complex animal viruses have been reported to show the presence of capsid-stabilizing proteins. It appears that during the course of evolution, viruses diverged to adopt various efficient ways for capsid stabilization, such as covalent bonding and the incorporation of decoration/stabilizing proteins [33] . The observation of protruding capsid proteins in Syn5 hints that such genes were likely acquired very early on for roles such as capsid stabilization, weak host cell surface recognition and host cell surface receptor mimicking. It has been suggested that phage/viral genes can travel laterally by several recombination events across wide phylogenetic distances—with different genes in the same phage often having different ancestry [46] . The sequence identities observed between knob-like proteins of Syn5 and the equivalence in other enteric phages, as well as some bacterial proteins, hint towards such lateral gene recombination events. The observation of capsid stabilizing proteins in Syn5 suggests the evolutionary significance of capsid stability/efficiency, where such genes were either acquired quite early on or more recently during virus evolution by means of lateral gene transfer. As the evolutionary age of marine viruses predates that of the enteric phages and animal viruses, it is possible that these structural features were acquired from the former during the course of evolution—although it may be a more recent phenomenon if these genes were acquired from the latter. Electron cryo-microscopy A sample of mature Syn5 virions was isolated and purified as described [5] . Briefly, Synechococcus WH8109 was grown to mid-log (in artificial sea water under constant light at 28 °C) and infected with a multiplicity of infection=0.001 phage per cell. On clearing, 1% CHCl 3 , 0.1% Triton X-100 and 0.01 mg ml −1 of lysozyme were added to complete lysis. The lysate of cell debris was removed by centrifugation and filtration. The phage was precipitated with 0.5 M NaCl and 10% PEG (8 K) stirring overnight in the cold. The precipitated phage was collected by centrifugation and resuspended in 50 mM Tris pH 7.5, 100 mM NaCl and 100 mM MgCl 2 . The suspension was loaded onto a CsCl step density gradient, the phage particles sedimented to the interface between ρ1.4 and ρ1.5. The resulting phage was concentrated by Vivaspin MWCO 100K (Sartorius). Aliquots of 2.7 μl of the purified phage sample were applied to glow-discharged (Gatan Plasma Cleaner) 400 mesh Quantifoil R1.2/1.3 copper grids (hole size 1.2 μm, Quantifoil Inc.), which were vitrified in liquid ethane by a FEI Vitrobot (MARK IV). Images of the frozen, hydrated sample were collected at a JEM3200FSC electron cryo-microscope (JEOL, Tokyo, Japan) operated at 300 keV at liquid nitrogen specimen temperature. The microscope is equipped with a field emission gun and an in-column omega energy filter (a slit width of 20 eV was used for data collection). The microscope settings include condenser aperture=50 μm, objective aperture=120 μm and spot size=1. The images were recorded on a Gatan 10K × 10K CCD camera, where 1,000 CCD frames were recorded at a nominal magnification of 80,000 (0.66 Å per pixel sampling rate), with a defocus range of 0.7–3.0 μm. The micrographs were computationally binned (2X) to obtain a final sampling of 1.32 Å in the images. Image processing and map validation Particles in various orientations were selected automatically using the swarm module in EMAN2 (ref. 47 ); the false-positive particles were deleted manually. This produced an initial data set of 18,000 particles. The contrast transfer function parameters for each CCD image were manually determined using ctfit in EMAN1 (ref. 8 ). An initial model was built from a small data set of 1,000 particles by assigning random orientations in multi-path simulated annealing [10] . The particle orientations were refined at an increasing resolution limit starting from 50 Å up to 10 Å. An iterative refinement was done until convergence to obtain the final map from ~12,000 particles. An FSC plot was obtained between the two maps generated from randomly split even/odd data sets. This FSC plot is called FSC data . To validate the map resolution and assess any noise overfitting during refinement, the method of HR noise substitution was used [11] , here the results are shown in Supplementary Fig. 1c . For this, a second stack from the original experimental data set was generated, where data beyond 10 Å was removed by randomizing the phases [11] . These HR noise-substituted data were then subjected to the identical protocol of 3D reconstruction as mentioned above for the experimental data. An FSC plot was obtained between the two maps generated from the randomly split even/odd HR noise data sets. This FSC plot is called FSC noise . In the HR noise-substituted data, the FSC drops significantly to zero past 10 Å, beyond which the data were substituted with noise, showing no significant noise overfitting (shaded blue area). An FSC true (black solid line) was plotted by calculating the relative error between the FSC data (pink dotted curve) and FSC noise (blue dotted curve), as described previously [10] . The true data with no overfitting are shaded pink in Supplementary Fig. 1c . The FSC true plot was used to estimate the resolution of the final map to be 4.7 Å at FSC=0.143. We applied experimentally determined structure factors [47] to the map for sharpening, limited to the reported resolution limit of 4.7 Å. Map visualization and analysis UCSF Chimera [48] was used for map visualization, analysis and generation of the molecular graphics images. The segmentation of the densities corresponding to the major capsid protein and the outer capsid proteins were done using Chimera and Avizo ( http://www.vsg3d.com/avizo/overview ). To generate an average of the six-hexameric subunits in one asymmetric unit for model building purposes, their corresponding densities were aligned in Foldhunter program [49] , while an average was calculated by proc3d in EMAN1. A pairwise FSC was calculated between the computationally segmented seven subunits in an asymmetric unit of the icosahedral map, where no symmetry is applied, to measure the correlation among the gp39 subunits within one asymmetric unit [50] . Sequence analysis and secondary structure prediction Various bioinformatic tools were used to analyse the sequences of gp39, gp55, gp57 and gp58 proteins. For the multiple sequence alignment and secondary structure prediction, PSIPRED [21] and Jpred [22] servers were used, while the physical and chemical parameters such as molecular weight, amino-acid composition, instability index, hydrophobicity and so on were calculated using ProtParam [23] and PredictProtein [24] servers. The knob proteins gp55/58 being farthest from the centre (highest alignment errors) are poorly resolved compared to the major capsid proteins, hence we have not built model for these proteins. Moreover, the capsid surface of Syn5 is thin and smoother as seen in Fig. 1a compared with other known phage structures such as ε15 and P22, hence fewer features to align at the extreme radius of the capsid shell. However, we were able to localize major SSEs using SSEHunter [25] in the map densities of gp55/gp58. Also, our analysis hints that the protruding density gp58 found at the opening of the hexamer is composed of two polypeptide chains. Model building and refinement for gp39 For model building, each of the seven individual gp39 subunits from one asymmetric subunit were cropped out of the full map using UCSF’s Chimera [48] . Individual gp39s were aligned with Foldhunter [49] and then averaged using proc3d, both of which are available in EMAN1 (ref. 8 ). Using the initial averaged gp39 density as a template, a second round of segmentation, alignment and averaging resulted in a final average gp39 subunit. SSE identification was then performed on the averaged gp39 subunit using SSEHunter in Gorgon 51 . Five helices and two β-sheets were identified and corresponded to those found in capsid proteins of other tailed dsDNA bacteriophages, such as gp5 in HK97 (ref. 14 ). In addition, a density skeleton was computed that revealed the topological linkages between the observed SSEs. Jpred 3.0 (ref. 22 ) was then used to predict the secondary structure from the sequence, also revealing five helices and several beta strands. Using Gorgon, an initial topology for gp39 was constructed by establishing a sequence to structure correspondence between the predicted and observed SSEs using the density skeleton as a constraint. From this topology, a Cα backbone model was then constructed using Gorgon’s semi-automated model building tools. Briefly, Cα backbone α-helices were first constructed in the density at the positions found by SSEHunter using the Helix editor function in the ‘semi-automatic atom placement’ utility in Gorgon. Loops between the α-helices were then built using Atom editor and Position editor functions in the ‘semi-automatic atom placement’ utility in Gorgon, which allows the user to place individual Cα backbone atoms along the density skeleton at a given spacing (~3.8 Å for Cα–Cα distances). Model building proceeded until the entire sequence of gp39 was placed within the density. Manual refinement of atom position was done interactively in Gorgon to remove any potential clashes and correct bad Cα–Cα distances. The final model was saved as a PDB file. To validate the model, we then used our Pathwalking protocol [17] to determine whether the solution found in Gorgon was unique. The initial Cα positions were iteratively perturbed (sigma=1) using e2pathwalker.py such that 100 potential model paths were computed with Pathwalker. For calculating these paths, the LKH TSP [17] solver was used. Results were examined and compared in UCSF’s Chimera [48] . A small amount of noise was added (sigma=1) to the positions of the initial Cα model using e2pathwalker.py from EMAN2. One hundred potential model paths were then computed using e2pathwalker.py and then compared in UCSF’s Chimera. In each case, the pathwalking model resulted in a continuous chain trace through the density map without any visible density crossovers. Topologically, all the models appeared similar with some differences occurring in the first ~25 amino acids. For the purposes of the remaining modelling, the first 25 amino acids were truncated from the model. Manual refinement of Cα positions was done interactively in Gorgon to correct bad Cα–Cα distances. In addition, COOT was used to remove clashes within and between subunits in the asymmetric unit. The final model was saved as a PDB file. Accession numbers A Cα backbone model of the major capsid protein gp39 of the mature virion of Syn5 has been deposited in the RCSB Protein Data Bank under accession code 4BMI . The original 3D cryo-EM density map has been deposited in the EMDataBank under accession code EMD-5954. How to cite this article: Gipson, P. et al . Protruding knob-like proteins violate local symmetries in an icosahedral marine virus. Nat. Commun. 5:4278 doi: 10.1038/ncomms5278 (2014).